Interplay between chemotaxis and contact inhibition of locomotion determines exploratory cell migration Directed cell migration in native environments is influenced by multiple migratory cues. These cues may include simultaneously occurring attractive soluble growth factor gradients and repulsive effects arising from cell–cell contact, termed contact inhibition of locomotion (CIL). How single cells reconcile potentially conflicting cues remains poorly understood. Here we show that a dynamic crosstalk between epidermal growth factor (EGF)-mediated chemotaxis and CIL guides metastatic breast cancer cell motility, whereby cells become progressively insensitive to CIL in a chemotactic input-dependent manner. This balance is determined via integration of protrusion-enhancing signalling from EGF gradients and protrusion-suppressing signalling induced by CIL, mediated in part through EphB. Our results further suggest that EphB and EGF signalling inputs control protrusion formation by converging onto regulation of phosphatidylinositol 3-kinase (PI3K). We propose that this intricate interplay may enhance the spread of loose cell ensembles in pathophysiological conditions such as cancer, and possibly other physiological settings. Directed cell migration is the ability of cells to orient their migration in response to diverse external cues. In native environments, cells often navigate in the context of multiple simultaneously presented cues, both attractive and repulsive, which jointly influence the activity and localization of migratory molecular networks. The concerted effects of multiple cues drive complex cellular behaviours, ultimately resulting in exquisite control of cell positioning and migration across considerable distances. Multiple migration cues are vital to developmental processes, such as topographic mapping in the visual system, where retinal ganglion cells are guided by attractive gradients of ephrins expressed on the surface of surrounding cells while experiencing a counterbalancing, repulsive gradient of soluble Wnt [1] . Another prominent example is the migration of neural crest cells in developing vertebrates, where guidance is achieved through recognition of several soluble cues, such as SDF-1, and mutual cell repulsion [2] , [3] . More generally, directionally migrating cells often need to resolve the effect of multiple inputs to make productive migration decisions. Understanding how single cells make such decisions remains challenging, in part, due to technological limitations complicating simultaneous delivery of several signalling inputs in a reliable manner, while observing the resulting intracellular signalling activities. Multiple cues also play a prominent role in influencing cell migration during pathological conditions, such as cancer metastasis. Metastatic cancer cells can enhance their responsiveness to migratory cues and overall locomotive capacity [4] through increased expression and activation of actin-binding proteins [5] , Rho-family GTPases [6] and receptor tyrosine kinases [7] . Various motile cues are provided by the tumour microenvironment, including soluble factors secreted by heterogeneous populations of stromal cells [8] and tumour-associated macrophages [9] , [10] , [11] . One prominent soluble cue is epidermal growth factor (EGF), a potent attractant shown to be critical for breast cancer chemotaxis both in vivo [12] and in vitro [13] . In addition to a progressive elucidation of the roles of soluble cues, recent work has rekindled interest in cell surface-bound cues, and, in particular, those mediating contact inhibition of locomotion (CIL), a phenomenon initially observed approximately 60 years ago by Abercrombie and Heaysman in fibroblasts [14] . CIL, in its most general description, is a suppression of forward locomotion on cell–cell contact and in many but not all cell types that display it, is followed by protrusion collapse and a subsequent redirection of cell motility. Interestingly, many malignant cells do not display CIL when interacting with other cell types (heterotypic), but retain CIL in interactions with each other (homotypic) [15] , [16] , [17] , [18] . These CIL characteristics may promote tumour invasiveness by preferentially directing cancer cells into the stromal environment [2] , [15] , [16] , [17] , with recent work pointing to an Eph receptor code as the molecular basis for this preferential CIL response in prostate cancer cells [17] . Although chemotaxis and CIL are now generally recognized as important regulators of directed cell migration during metastasis, the interactions between these cues and how cancer cells integrate them are still poorly understood. In particular, it is unclear how cells choose the direction of their migration in situations where different cues simultaneously act to specify opposing directions of motility and how the resulting decisions may affect the behaviour of the cell population. Here we investigate the interplay between CIL and chemotaxis using MTLn3 rat breast adenocarcinoma cells overexpressing the epidermal growth factor receptor (EGFR) and GFP, referred to as MTLn3-B1 (ref. 7 ). These cells are highly metastatic [7] , exhibiting enhanced chemotaxis to EGF in vitro and in vivo and display a qualitatively similar CIL response to fibroblasts, where contact between the leading processes of two cells results in a suppression of forward migration, a collapse of protrusions and a switch in polarity [19] . Using a new microfluidic-device-based assay that allows a controlled, direct comparison of the effects of chemotactic and CIL cues at the single cell level, we explore the molecular mediators of these cues in MTLn3-B1 cells. We find that the outcome of integration of chemotaxis and CIL is determined by a dose-dependent balance between the intracellular signalling processes triggered by these cues. We suggest that the interplay between these cues can serve to switch between random and directed invasive cell migration, while serving as a more general paradigm for how other cellular systems resolve multiple cues. MTLn3-B1 cell chemotaxis varies across EGF gradients To quantitatively assay the effects of EGF gradients and to enhance the probability of cell–cell interactions leading to CIL, we developed a new microfluidic device based on previously developed device architectures [20] , [21] , whereby gradients of soluble factors are generated across parallel arrays of cell-laden microchannels ( Fig. 1a ). These gradients develop across the microchannels via passive diffusion between a continually replenished source and sink, and can be dynamically controlled by pneumatic valves, eliminating the latency in gradient development between the first and last channel in the array ( Supplementary Fig. 1 , See Methods for more details). Cell migration within the microchannels is constrained to one dimension, due to the limited cross-section of the microchannels (14 μm by 6 μm, width by height). This one dimensional motility optimizes the opportunities for CIL events to occur between closely positioned migrating cells (similar to the effects of micropatterned cell adhesion substrata [22] , [23] ), while also providing an unambiguous readout of both chemotactic guidance and cell collision outcomes based on the resulting direction of cell migration. Moreover, this migration pattern mimics some of the topological features of cancer cell migration in vivo , where cancer cells migrate along collagen fibres in sparser regions of matrix [24] or through spatially confined tunnels of degraded matrix [25] . 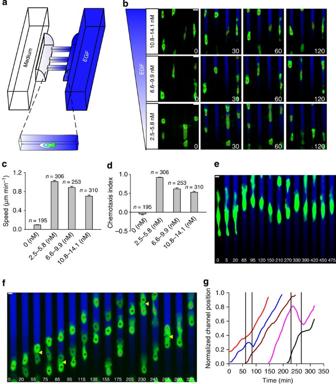Figure 1: MTLn3-B1 chemotaxis in different EGF gradients and influences from CIL. (a) Schematic of the microfluidic device used to produce defined gradients of EGF across microchannels housing MTLn3-B1 cells. (b) Representative images of MTLn3-B1 cells undergoing chemotaxis in different EGF gradients. Green colour visualizes expression of GFP. The gradient is visualized with a Dextran dye shown in blue here and in subsequent images. Red asterisks track cell positions from time=0. Images are rotated to aid in visualization. Times are in minutes. Scale bar, 20 μm. (c,d) Quantification of velocity and chemotaxis index of MTLn3-B1 cells under control (0 nM) and indicated EGF gradients from (b). Data are the mean from the number of indicated cells fromn>=3 independent experiments with error bars showing s.e.m. (e) An MTLn3-B1 cell displaying oscillations in migration in 10.8–14.1 nM EGF gradients. (f) MTLn3-B1 cells undergoing CIL during chemotaxis. Coloured asterisks track different cells. Yellow arrows highlight CIL events. Time is in minutes. Scale bar, 10 μm. (g) Quantification of channel position of MTLn3-B1 cells in (f). Coloured lines track the position of the corresponding cells in (g) denoted by similarly coloured asterisks. Black vertical lines indicate collisions. Figure 1: MTLn3-B1 chemotaxis in different EGF gradients and influences from CIL. ( a ) Schematic of the microfluidic device used to produce defined gradients of EGF across microchannels housing MTLn3-B1 cells. ( b ) Representative images of MTLn3-B1 cells undergoing chemotaxis in different EGF gradients. Green colour visualizes expression of GFP. The gradient is visualized with a Dextran dye shown in blue here and in subsequent images. Red asterisks track cell positions from time=0. Images are rotated to aid in visualization. Times are in minutes. Scale bar, 20 μm. ( c , d ) Quantification of velocity and chemotaxis index of MTLn3-B1 cells under control (0 nM) and indicated EGF gradients from ( b ). Data are the mean from the number of indicated cells from n >=3 independent experiments with error bars showing s.e.m. ( e ) An MTLn3-B1 cell displaying oscillations in migration in 10.8–14.1 nM EGF gradients. ( f ) MTLn3-B1 cells undergoing CIL during chemotaxis. Coloured asterisks track different cells. Yellow arrows highlight CIL events. Time is in minutes. Scale bar, 10 μm. ( g ) Quantification of channel position of MTLn3-B1 cells in ( f ). Coloured lines track the position of the corresponding cells in ( g ) denoted by similarly coloured asterisks. Black vertical lines indicate collisions. Full size image We first assessed how freely migrating MTLn3-B1 cells would respond to different gradients of EGF with a constant concentration difference (3.3 nM) and varied mean concentrations (4.1, 8.3 and 12.4 nM ) ( Fig. 1b and Supplementary Movie 1 ). On introduction of EGF gradients, we observed the formation of large cell protrusions towards the source of EGF and rapid cell motility up the gradient ( Fig. 1b ). MTLn3-B1 cells displayed the highest speed and greatest accuracy in 2.5–5.8 nM EGF gradients, rarely changing directions and maintaining constant speeds ( Fig. 1c,d and Supplementary Movie 1 ). In contrast, cells remained relatively stationary without a preferential direction in medium devoid of EGF ( Fig. 1c,d , Supplementary Fig. 2a ). Cell speed and accuracy decreased with increasing mean EGF concentration, but still retained a net preference up the gradient ( Fig. 1b–d ). In particular, in gradients with a high mean EGF concentration (10.8–14.1 nM gradient, 12.4 nM mean concentration), many MTLn3-B1 cells displayed elongated cell morphologies and oscillatory migration, with a frequent collapse of leading protrusions ( Fig. 1e ). Increases in the gradient steepness (6.6 nM concentration difference across channels, 5.0–11.6 nM EGF) did not enhance chemotactic bias beyond the values found in the optimal gradient determined above (2.5–5.8 nM EGF) ( Supplementary Fig. 2b–d ). EGFR overexpression in MTLn3 cells has been previously associated with an increase in overall motility, augmented chemotaxis and an enhanced metastatic potential [7] . Therefore, to validate our assay, we next investigated EGF chemotaxis in native MTLn3 cells ( Supplementary Fig. 3 ). Similar to MTLn3-B1 cells, MTLn3 cells displayed little motility in the absence of EGF ( Supplementary Fig. 3a ). MTLn3 cells exhibited clear chemotaxis in 2.5–5.8 nM gradients of EGF, but had decreased speed and accuracy, as compared with MTLn3-B1 cells ( Fig. 1c,d , Supplementary Fig. 3b,d,e ), in agreement with previous results [7] . In sharper EGF gradients (6.6 nM concentration difference, 5.0–11.6 nM EGF gradient), MTLn3 cell accuracy did not improve but cell speed increased ( Supplementary Fig. 3c–e ). Taken together, our results indicate that MTLn3 cells can undergo effective chemotaxis in EGF gradients, with response precision limited by the total ambient EGF concentration and EGFR expression. We next analysed how CIL affects chemotaxis by observing the direction of motility of cell pairs after a collision. If CIL occurs equally, a given cell collision would result in a pairwise halt in migration, a collapse of protrusions, and redirection. Interestingly, we frequently observed non-reciprocal CIL interactions where only a single member of the colliding cell pair was redirected, resulting in ‘ping pong’ migration patterns induced by sequential cell–cell collisions. ( Fig. 1f,g , Supplementary Movie 2 ). These results suggested that the choice between continual migration and redirection in the presence of chemical gradients and cell–cell contact likely depends strongly, albeit stochastically, on chemotactic input, prompting us to further quantitatively explore the interplay between chemotactic and CIL signalling. CIL occurs in an EGF dose-independent manner We began by characterizing the baseline CIL behaviour in MTLn3-B1 cells within microchannels in different uniform concentrations of EGF (4.1, 8.3 and 12.4 nM), matching the mean EGF concentrations of the gradients analysed above. In the presence of uniform EGF, MTLn3-B1 cells displayed frequent switches in migration direction and recurrent CIL events ( Fig. 2a ). Cell collisions were classified into one of two categories according to whether a leading cell protrusion in one of the colliding cells interacted with the leading protrusion in the second cell (termed ‘head-to-head’ (HH) collision) or with the trailing edge of the second cell (termed ‘head-to-tail’ (HT) collision). We found that three different outcomes arose from a HH collision ( Fig. 2b and Supplementary Movie 3 ), depending on whether CIL occurred in a single member of the cell pair (Outcome 1, 3) or in both (Outcome 2), with the outcome occurring probabilistically, as suggested previously [23] . Protrusions typically collapsed and reformed in a span of 15–35 min after initial contact between colliding cells across all tested EGF concentrations, with a maximum observed duration of 60 min ( Supplementary Fig. 4a ). The majority of HH collisions lead to the repulsion of both cells (Outcome 2), irrespective of the EGF dose ( Fig. 2c ), suggesting a predominantly equal CIL effect in cell pairs under uniform EGF. In HH collisions where cells did not switch polarity (Outcome 1 or Outcome 3), the protrusions of these cells remained unaffected by the collision ∼ 30% of the time, independent of the original direction of migration ( Supplementary Fig. 4b,c ), suggesting the stochastic presence of a more stable population of protrusions. In HT collisions, two distinct outcomes were observed, characterized by whether CIL did not (Outcome 1) or did (Outcome 2) occur ( Fig. 2d and Supplementary Movie 4 ). These collisions primarily resulted in repulsion of the trailing cell without affecting the leading cell (Outcome 2), also in an EGF dose-independent manner ( Fig. 2e ). CIL propensities were similar in MTLn3 cells under uniform EGF ( Supplementary Fig. 3f,g ), indicating that overexpression of EGFR does not influence CIL. 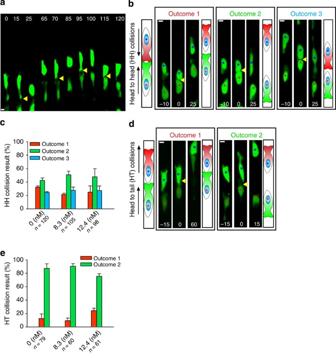Figure 2: Characterization of CIL in uniform concentrations of EGF. (a) MTLn3-B1 cells displaying random motility and undergoing multiple CIL events in a uniform concentration of EGF (8.3 nM ). (b,d) Representative examples of the outcomes of head-to-head and head-to-tail collisions in MTLn3-B1 cells with corresponding illustrations, respectively. Collisions occur at timet=0. Coloured asterisks track different cells. Yellow arrows indicate collisions. Time is in minutes. Scale bar, 10 μm. (c,e) Probability of head-to-head and head-to-tail collision outcomes in the indicated uniform concentrations of EGF. The total number of cells are indicated per condition. Data represent the mean fromn=3 independent experiments per condition and error bars show s.e.m. Figure 2: Characterization of CIL in uniform concentrations of EGF. ( a ) MTLn3-B1 cells displaying random motility and undergoing multiple CIL events in a uniform concentration of EGF (8.3 nM ). ( b , d ) Representative examples of the outcomes of head-to-head and head-to-tail collisions in MTLn3-B1 cells with corresponding illustrations, respectively. Collisions occur at time t =0. Coloured asterisks track different cells. Yellow arrows indicate collisions. Time is in minutes. Scale bar, 10 μm. ( c , e ) Probability of head-to-head and head-to-tail collision outcomes in the indicated uniform concentrations of EGF. The total number of cells are indicated per condition. Data represent the mean from n =3 independent experiments per condition and error bars show s.e.m. Full size image Cells experiencing CIL in open two-dimensional environments typically have several degrees of freedom to reinitiate migration. Our assay substantially reduced the free space available for cell migration after cell–cell collisions, potentially altering native CIL behaviour. Therefore, we next investigated whether MTLn3-B1 cells also display CIL in a dose-independent manner in 2D environments using a different microfluidic device and quantified CIL using previously established CIL metrics [17] , [18] ( Supplementary Fig. 5 ) (See Methods for description of analysis). Similar to our results in 1D ( Fig. 2c,e ), MTLn3-B1 cells also exhibited CIL in 2D environments in an EGF dose-independent manner ( Supplementary Fig. 5e ). Overall, our results demonstrate that CIL responses are largely independent of ambient, uniform EGF concentrations. Integration of chemotaxis and CIL is input dependent As uniform EGF exposure did not affect the probabilistic outcomes of CIL, we next investigated whether the effect of EGF on CIL outcomes would depend on spatially graded EGF presentation ( Fig. 3a ). In a 2.5–5.8 nM EGF gradient, found to be optimal for MTLn3-B1-directed migration ( Fig. 1b–d ), we detected a significant shift in HH CIL probabilities towards outcome 1 (CIL occurs solely in cells initially migrating away from the gradient (blue asterisk)), as compared with the corresponding, uniform 4.1 nM EGF dose ( Fig. 3b,c , Supplementary Movie 5 ), indicating that optimal chemotactic signalling strongly overrides CIL. This change was diminished but still significant in 6.6–9.9 nM EGF gradients as compared with the uniform 8.3 nM EGF dose ( Fig. 3d ), but was completely lost in the 10.8–14.1 nM EGF gradient ( Fig. 3e ), where the collision outcomes mirrored those found in the uniform 12.4 nM EGF dose. Protrusions collapsed and reformed after initial contact on a similar timescale in gradients of EGF as compared with uniform EGF, with a moderate shift towards longer durations in 10.8–14.1 nM EGF gradients ( Supplementary Fig. 4d ), suggesting that EGF gradients do not significantly affect temporal aspects of CIL interactions. However, cell protrusions oriented towards optimal EGF gradients became substantially more stable, as such protrusions were more than twice as likely to remain unaffected by collisions as compared with protrusions in uniform EGF ( ∼ 80% versus ∼ 30%, Supplementary Fig. 4e , Fig. 3f ), while protrusions oriented away from EGF gradients behaved similarly ( Supplementary Fig. 4f ). A similar gradient-dependent shift in CIL probabilities also occurred in HT collisions ( Fig. 3g , Supplementary Movie 6 ), with trailing cells (red asterisk) failing to undergo CIL (outcome 1) after collisions with leading cells (blue asterisk) in optimal EGF gradients ( Fig. 3h–j ). The net result of this switch was the appearance of co-migrating cell clusters ( Fig. 3k ), resembling cellular streaming behaviour seen in MTLn3 migration in vivo [7] . Collision outcomes in MTLn3 cells in 2.5–5.8 nM EGF gradients showed similar biases ( Supplementary Fig. 3f,g ), albeit less strong than those seen in MTLn3-B1 cells ( Fig. 3c,h ), suggesting that EGFR overexpression reduces the probability of CIL during chemotaxis. Overall, our results suggest that modulating the strength of chemotactic behaviour, either by altering external gradient inputs or by changing receptor expression, can dynamically alter the balance between chemotaxis and CIL cues. 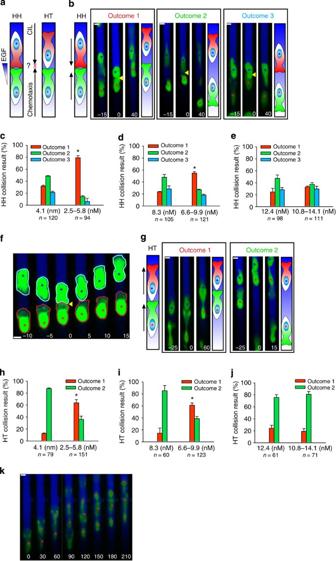Figure 3: Integration of chemotaxis and CIL is input dependent. (a) Schematic of how chemotaxis and CIL cues conflict during different cell collisions. (b,g) Examples of the outcomes of head-to-head (b) and head-to-tail (g) collisions in MTLn3-B1 cells in gradients of EGF with corresponding illustrations. Collisions occur at timet=0. Green colour indicates expression of GFP. The gradient of EGF is shown in blue visualized with a Dextran dye here and in all subsequent images. Coloured asterisks track different cells. Yellow arrows indicate collisions. (c–e) Probabilities of head-to-head collision outcomes in gradients of EGF versus uniform concentrations. Uniform concentrations are taken fromFig. 2c. Number of collisions analysed is indicated. Data shown are the mean ofn=3 independent experiments with error bars representing s.e.m.. Statistical comparisons are made between the same outcome (red bars) in uniform versus gradient using a two-sided student’st-test. (f) Example of a head-to-head collision in which the protrusion of an MTLn3-B1 cell migrating up the gradient (red outline, red asterisk) is not affected by a cell collision (other colliding cell shown with blue outline, blue asterisk). Timet=0 denotes when the collision occurred. Yellow arrow indicates the collision. (h–j) Probabilities of head-to-tail collision outcomes in gradients of EGF versus uniform concentrations. Uniform concentrations are taken fromFig. 2e. Total collisions analysed per condition are displayed. Data are the mean ofn=3 independent experiments per condition. Error bars are s.e.m.. Statistical comparisons are made between the same outcome (red bars) in uniform versus gradient using a two-sided student’st-test. (k) A group of MTLn3-B1 cells streaming up a gradient of EGF. Red asterisks track cell positions. Time is in minutes. Scale bar, 10 μm. *P<1e−3. Figure 3: Integration of chemotaxis and CIL is input dependent. ( a ) Schematic of how chemotaxis and CIL cues conflict during different cell collisions. ( b , g ) Examples of the outcomes of head-to-head ( b ) and head-to-tail ( g ) collisions in MTLn3-B1 cells in gradients of EGF with corresponding illustrations. Collisions occur at time t =0. Green colour indicates expression of GFP. The gradient of EGF is shown in blue visualized with a Dextran dye here and in all subsequent images. Coloured asterisks track different cells. Yellow arrows indicate collisions. ( c – e ) Probabilities of head-to-head collision outcomes in gradients of EGF versus uniform concentrations. Uniform concentrations are taken from Fig. 2c . Number of collisions analysed is indicated. Data shown are the mean of n =3 independent experiments with error bars representing s.e.m.. Statistical comparisons are made between the same outcome (red bars) in uniform versus gradient using a two-sided student’s t -test. ( f ) Example of a head-to-head collision in which the protrusion of an MTLn3-B1 cell migrating up the gradient (red outline, red asterisk) is not affected by a cell collision (other colliding cell shown with blue outline, blue asterisk). Time t =0 denotes when the collision occurred. Yellow arrow indicates the collision. ( h – j ) Probabilities of head-to-tail collision outcomes in gradients of EGF versus uniform concentrations. Uniform concentrations are taken from Fig. 2e . Total collisions analysed per condition are displayed. Data are the mean of n =3 independent experiments per condition. Error bars are s.e.m.. Statistical comparisons are made between the same outcome (red bars) in uniform versus gradient using a two-sided student’s t -test. ( k ) A group of MTLn3-B1 cells streaming up a gradient of EGF. Red asterisks track cell positions. Time is in minutes. Scale bar, 10 μm. * P <1e−3. Full size image Taken together, the results above suggested that chemotaxis and CIL individually regulated signalling at cell protrusions, with chemotactic and CIL signalling providing positive and negative regulation, respectively. However, it still remained unclear whether this regulation is achieved through independent parallel pathways converging on cytoskeletal components found in leading protrusions or through regulation of upstream shared signalling components. Therefore, we next set out to clarify the roles of molecular components involved in chemotaxis and CIL signalling in MTLn3-B1 cells. Chemotaxis signalling in MTLn3-B1 cells PI3K and the small Rho GTPase, Rac, have been strongly implicated in chemotaxis and are active at the leading protrusions of many chemotactic cells, such as amoebae cells [26] , [27] , neutrophils [28] , [29] and fibroblasts [30] , [31] . In MTLn3 cells, PI3K and Rac activities rapidly increase at protrusions after uniform EGF stimulation, peaking at ∼ 1 min and returning to baseline within several minutes [32] . However, the activity of these molecules in live MTLn3 cells during long-term exposure to EGF gradients has not been explored. Therefore, we transfected MTLn3-B1 cells with PI3K and Rac biosensors and observed their responses during EGF chemotaxis. To monitor PI3K activity, we used a mCherry-tagged pleckstrin homology (PH) domain of Akt (mCH-Akt-PH) ( Fig. 4a ), determining its ratio to cyotosolic GFP to account for possible volume alteration effects [33] . PI3K activity became locally enriched at the cell front in EGF gradients ( Fig. 4a and Supplementary Movie 7 ), with a peak of activity at 6 min ( Fig. 4b ) followed by decreased but sustained activity. Conversely, a control mCherry construct without a PH domain did not show any polarization ( Fig. 4b , Supplementary Fig. 6a ). Rac also became locally activated at the cell front in EGF gradients ( Fig. 4c and Supplementary Movie 8 ), as assessed with a Raichu-Rac FRET sensor [34] , but with slower kinetics ( Fig. 4d ). In the absence of EGF, cells did not generate protrusions and Rac activity remained unpolarized ( Fig. 4d , Supplementary Fig. 6b ). Analysis of a RFP-tagged Lifeact [35] sensor confirmed that chemotaxing MTLn3-B1 cells migrate in this assay via the generation of F-actin-rich protrusions ( Fig. 4e ). Overall, we find that PI3K and Rac become polarized and retain persistent activity at the front of MTLn3-B1 cells during EGF chemotaxis over at least a 40-min period, and thus highlight differential regulation of activity under uniform versus graded stimulation in MTLn3 cells. 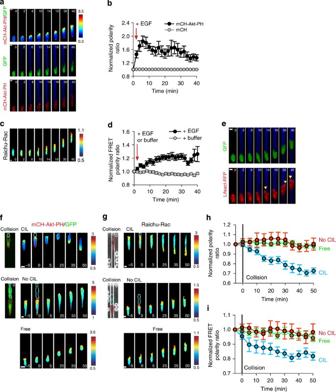Figure 4: PI3K and Rac polarize and retain persistent activity at the leading edge during chemotaxis and are inhibited during CIL. (a) Representative images of PI3K activity during MTLn3-B1 chemotaxis to EGF (2.5–5.8 nM). The pseudcolour images (top panel) represent the ratio between mCH-Akt-PH and GFP. The green colour (middle panel) visualizes GFP expression. Red colour (bottom panel) displays mCH-Akt-PH. (b) Quantification of the polarity ratio in chemotaxing mCH-Akt-PH-expressing MTLn3-B1 cells versus control mCH-expressing cells. Data represent the mean ofn>=20 cells per condition fromn=3 independent experiments. Error bars are s.e.m. (c) Representative images of Rac activity during MTLn3-B1 chemotaxis to EGF (2.5–5.8 nM). Pseudocolour images show the FRET ratio (YFP FRET/CFP) from a Raichu-Rac construct. (d) Quantification of the FRET polarity ratio in MTLn3-B1 cells with and without a gradient of EGF. Data represent the mean fromn>=12 cells fromn=3 independent experiments. Error bars show s.e.m. (e) Representative images of the localization of F-actin during MTLn3-B1 chemotaxis to EGF (2.5–5.8 nM). Green colour (top panel) indicates expression of GFP. Red colour (bottom panel) displays Lifeact-RFP. Yellow arrows highlight localized enrichment of F-actin. (f,g) Visualization of (f) PI3K activity and (g) Rac activity in cells in collisions resulting in CIL (top panel), not resulting in CIL (middle panel), and in freely migrating cells (bottom panel). Collisions occur at timet=0. The first image in the top and middle series of images visualizes the collision, showing the tracked cell outlined in red and the cell it is colliding with in blue. These outlines are reproduced in the ratio image at timet=0. Pseudocolour images represent the ratio between mCH-Akt-PH and GFP in (f) and the FRET ratio (YFP FRET/CFP) in (g). (h,i) Quantification of the polarity ratio in cells in collisions with and without CIL and free moving cells for (h) PI3K and (i) Rac. Data represent the mean fromn>=11 cells per condition from three independent experiments with error bars representing s.e.m. Time is in minutes. Scale bar, 10 μm. Figure 4: PI3K and Rac polarize and retain persistent activity at the leading edge during chemotaxis and are inhibited during CIL. ( a ) Representative images of PI3K activity during MTLn3-B1 chemotaxis to EGF (2.5–5.8 nM). The pseudcolour images (top panel) represent the ratio between mCH-Akt-PH and GFP. The green colour (middle panel) visualizes GFP expression. Red colour (bottom panel) displays mCH-Akt-PH. ( b ) Quantification of the polarity ratio in chemotaxing mCH-Akt-PH-expressing MTLn3-B1 cells versus control mCH-expressing cells. Data represent the mean of n >=20 cells per condition from n =3 independent experiments. Error bars are s.e.m. ( c ) Representative images of Rac activity during MTLn3-B1 chemotaxis to EGF (2.5–5.8 nM). Pseudocolour images show the FRET ratio (YFP FRET/CFP) from a Raichu-Rac construct. ( d ) Quantification of the FRET polarity ratio in MTLn3-B1 cells with and without a gradient of EGF. Data represent the mean from n >=12 cells from n =3 independent experiments. Error bars show s.e.m. ( e ) Representative images of the localization of F-actin during MTLn3-B1 chemotaxis to EGF (2.5–5.8 nM). Green colour (top panel) indicates expression of GFP. Red colour (bottom panel) displays Lifeact-RFP. Yellow arrows highlight localized enrichment of F-actin. ( f , g ) Visualization of ( f ) PI3K activity and ( g ) Rac activity in cells in collisions resulting in CIL (top panel), not resulting in CIL (middle panel), and in freely migrating cells (bottom panel). Collisions occur at time t =0. The first image in the top and middle series of images visualizes the collision, showing the tracked cell outlined in red and the cell it is colliding with in blue. These outlines are reproduced in the ratio image at time t =0. Pseudocolour images represent the ratio between mCH-Akt-PH and GFP in ( f ) and the FRET ratio (YFP FRET/CFP) in ( g ). ( h , i ) Quantification of the polarity ratio in cells in collisions with and without CIL and free moving cells for ( h ) PI3K and ( i ) Rac. Data represent the mean from n >=11 cells per condition from three independent experiments with error bars representing s.e.m. Time is in minutes. Scale bar, 10 μm. Full size image We next assessed whether PI3K and Rac activities at cell protrusions were regulated by CIL by observing their activity in cell collisions where CIL did and did not occur, with single, freely chemotaxing MTLn3-B1 cells as controls ( Fig. 4f,g ). Both freely chemotaxing MTLn3-B1 cells and colliding cells that did not display CIL maintained constant PI3K and Rac activities at the cell front, whereas in cell collisions where CIL did occur, PI3K and Rac were locally inhibited at the contacting leading edge during its collapse ( Fig. 4f–i and Supplementary Movies 9,10 ). PI3K and Rac activities then relocalized to the opposite end of cells, coincident with the formation of a new protrusion and initiation of cell migration in the new direction ( Fig. 4h,i and Supplementary Movies 9,10 ). These results suggested that, for CIL to occur, PI3K and Rac must be locally downregulated at the point of cell contact and prompted us to explore the molecular mediators of CIL signalling in MTLn3-B1 cells. Eph B signalling induces CIL in MTLn3-B1 cells CIL in MTLn3-B1 cells could potentially be mediated by the physical obstruction of space available for formation and adhesion of cell protrusions rather than through active interfacial cell–cell signalling. To address this possibility, we introduced 3T3 fibroblasts into microchannels with MTLn3-B1 cells. EGF gradients induced cancer cell migration without affecting fibroblast motility, thus leading to cancer cell–fibroblast collisions ( Fig. 5a ). Although 3T3 cells encompassed most of the microchannel, we found that the majority of chemotaxing MTLn3-B1 cells could migrate around and actively displace the fibroblast cells (9/10 collisions result in migration past 3T3 cells) ( Fig. 5b and Supplementary Movie 11 ), indicating reduced heterotypic CIL. This result suggested that physical hindrance is unlikely to account for CIL in MTLn3-B1 cells, as the mechanical properties of fibroblasts are expected to be similar to those of MTLn3-B1 cells, and further implied that active cell-to-cell signalling is likely to mediate CIL. 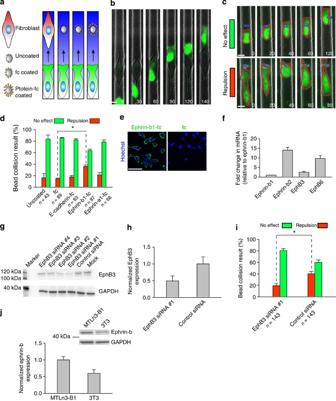Figure 5: EphB signalling is sufficient to induce CIL in MTLn3-B1 cells. (a) Schematic of the different obstacles assessed for their ability to induce CIL in chemotaxing MTLn3-B1 cells (2.5–5.8 nM EGF gradients). (b) An MTLn3-B1 cell migrating around a 3T3 cell during chemotaxis. Green colour indicates expression of GFP in the MTLn3-B1 cell. (c) Examples of MTLn3-B1 cells undergoing repulsion (top panel) or being unaffected (bottom panel) by collisions with silica beads during EGF chemotaxis. Red dashed lines highlight cell boundaries. Blue dashed lines outline silica beads. Time is in minutes. Scale bar, 10 μm. (d) Quantification of MTLn3-B1 bead collision events during chemotaxis with different silica bead coatings. Number of total collisions analysed per condition is indicated fromn>=2 independent experiments per condition. Error bars are s.e.m. Statistical comparisons are assessed with a two-sided Student’st-test. *P<.05. (e) Visualization of the binding of ephrin-b1-fc or fc to cells by immunostaining against the fc domain (shown in green). Nuclei are denoted in blue with Hoechst 33342. Scale bar, 50 μm. (f) Relative expression of ephrin-b ligand and EphB receptors in MTLn3-B1 cells from real-time RT-PCR. Data represent the mean fromn=3 biological replicates. Error bars are s.d. (g) Representative western blot of four different siRNA knockdowns of EphB3 in MTLn3-B1 cells along with control siRNA (non targeting) and mock-treated cells. GAPDH is the loading control. (h) Quantification of EphB3 knockdown in MTLn3-B1 cells using EphB3 siRNA #1 compared with a control siRNA. Data are from three independent experiments and are normalized to a loading control (GAPDH). Errors bars are s.d. (i) Quantification of collision results between EphB3 siRNA#1-treated or control siRNA-treated MTLn3-B1 cells with ephrin-b1-fc-coated beads. Number of total collisions analysed per condition is indicated fromn=3 independent experiments. Error bars are s.e.m. Statistical comparisons are assessed with a two-sided Student’st-test. *P<.05. (j) Quantification of ephrin-b isoforms in MTLn3-B1 cells and 3T3 cells. Data are taken fromn=3 independent replicates. (Inset) Representative western blot of ephrin-b isoforms in MTLn3-B1 cells and 3T3 cells. GAPDH is used as a loading control. Figure 5: EphB signalling is sufficient to induce CIL in MTLn3-B1 cells. ( a ) Schematic of the different obstacles assessed for their ability to induce CIL in chemotaxing MTLn3-B1 cells (2.5–5.8 nM EGF gradients). ( b ) An MTLn3-B1 cell migrating around a 3T3 cell during chemotaxis. Green colour indicates expression of GFP in the MTLn3-B1 cell. ( c ) Examples of MTLn3-B1 cells undergoing repulsion (top panel) or being unaffected (bottom panel) by collisions with silica beads during EGF chemotaxis. Red dashed lines highlight cell boundaries. Blue dashed lines outline silica beads. Time is in minutes. Scale bar, 10 μm. ( d ) Quantification of MTLn3-B1 bead collision events during chemotaxis with different silica bead coatings. Number of total collisions analysed per condition is indicated from n >=2 independent experiments per condition. Error bars are s.e.m. Statistical comparisons are assessed with a two-sided Student’s t -test. * P <.05. ( e ) Visualization of the binding of ephrin-b1-fc or fc to cells by immunostaining against the fc domain (shown in green). Nuclei are denoted in blue with Hoechst 33342. Scale bar, 50 μm. ( f ) Relative expression of ephrin-b ligand and EphB receptors in MTLn3-B1 cells from real-time RT-PCR. Data represent the mean from n =3 biological replicates. Error bars are s.d. ( g ) Representative western blot of four different siRNA knockdowns of EphB3 in MTLn3-B1 cells along with control siRNA (non targeting) and mock-treated cells. GAPDH is the loading control. ( h ) Quantification of EphB3 knockdown in MTLn3-B1 cells using EphB3 siRNA #1 compared with a control siRNA. Data are from three independent experiments and are normalized to a loading control (GAPDH). Errors bars are s.d. ( i ) Quantification of collision results between EphB3 siRNA#1-treated or control siRNA-treated MTLn3-B1 cells with ephrin-b1-fc-coated beads. Number of total collisions analysed per condition is indicated from n =3 independent experiments. Error bars are s.e.m. Statistical comparisons are assessed with a two-sided Student’s t -test. * P <.05. ( j ) Quantification of ephrin-b isoforms in MTLn3-B1 cells and 3T3 cells. Data are taken from n =3 independent replicates. (Inset) Representative western blot of ephrin-b isoforms in MTLn3-B1 cells and 3T3 cells. GAPDH is used as a loading control. Full size image To more specifically assay potential mediators of CIL in MTLn3-B1 cells, we utilized Protein A-coated silica beads, which can be functionalized with fc-tagged proteins and thus can be used to screen for specific proteins that may induce CIL [17] ( Fig. 5a ). We first assessed cell collisions with uncoated beads, detecting a number of repulsion events ( Fig. 5c,d and Supplementary Movie 12 ); however, the majority of cell-bead collisions did not affect the directionality of MTLn3-B1 cell migration, further supporting the relatively low importance of the effect of physical obstacles in CIL ( Fig. 5d ). Coating beads solely with the fc domain induced cell repulsion with equal probability to that found for uncoated protein A beads, indicating that the fc domain itself did not provide any signalling ( Fig. 5d ). As a first potential CIL mediator we tested E-cadherin, as cadherins have been implicated in CIL in Xenopus laevis neural crest cells [2] and quail myoblasts [36] . Furthermore, E-cadherin was previously shown to be upregulated in metastatic MTLn3 cells versus nonmetastatic variant MTC cells [9] and could be readily detected with immunostaining ( Supplementary Fig. 7a ). However, we found that E-cadherin-fc-coated silica beads did not significantly increase repulsion of chemotaxing MTLn3-B1 cells ( Fig. 5d ). We next examined the potential role of Eph receptors known to mediate repulsion in a diverse set of cells, such as axons [37] , prostate cancer cells [17] and endothelial cells [38] . Eph receptors are the largest family of receptor tyrosine kinases [39] and can be divided into A and B families based on their affinity for glycosylphospatidylinositol-linked ephrin-a or transmembrane ephrin-b ligands [40] . To investigate whether Eph receptor signalling was sufficient to induce CIL in chemotaxing MTLn3-B1 cells, we functionalized beads with either ephrin-b1-fc or ephrin-a1-fc, which can promiscuously bind EphB and EphA receptors [41] , respectively. We found that ephrin-b1-fc, but not ephrin-a1-fc, coated beads resulted in a twofold increase in the probability of contact repulsion with MTLn3-B1 cells ( Fig. 5d ), suggesting that EphB signalling contributes to the induction of CIL. We verified the presence of EphB receptors on MTLn3-B1 cells by incubating live MTLn3-B1 cells with various unclustered soluble ephrin-b-fc ligands and immunostaining for the fc domain ( Fig. 5e , Supplementary Fig. 7b ). Incubation with the fc domain itself did not produce any signal, indicating that the binding of the ephrin-b ligands was specific to their substrates, the EphB receptors ( Fig. 5e ). We also confirmed that MTLn3-B1 cells express EphA receptors by incubation and subsequent immunostaining with various ephrin-a-fc ligands ( Supplementary Fig. 7c ). Real-time RT-PCR further verified the expression of various ephrin-b and EphB transcripts in MTLn3-B1 cells ( Fig. 5f ). Ephrin-b2 was the predominant ephrin-b isoform, displaying similar cell surface binding to that of ephrin-b1 ( Fig. 5e , Supplementary Fig. 7b ), suggesting that both ephrin-b ligands can bind EphB receptors on MTLn3-B1 cells with similar affinity. To provide a causal role for EphB signalling in inducing CIL, we knocked down the EphB3 receptor in MTLn3-B1 cells using siRNA ( Fig. 5g ) and ran collision experiments between EphB3 knockdown MTLn3-B1 cells and ephrin-b1-fc-coated beads. We targeted the EphB3 receptor due to the known mutations in the EphB6 receptor that render it kinase null [40] . The siRNA with the greatest efficacy achieved ∼ 50% EphB3 depletion ( Fig. 5h ) and was chosen for further experimentation. We found a significant difference between the repulsion probabilities of EphB3 knockdown and control cells ( Fig. 5i ); specifically, knockdown of the EphB3 receptor decreased the probability of repulsion when encountering ephrin-b1-fc-coated beads ( Fig. 5i ) to a level comparable to the probabilities observed for untreated MTLn3-B1 cells encountering uncoated and fc-coated beads ( Fig. 5d ), while MTLn3-B1 cells treated with a control siRNA were repelled from ephrin-b1-fc-coated beads with a similar probability as untreated cells ( Fig. 5i ), supporting a role for EphB3 signalling in inducing CIL in MTLn3-B1 cells. Last, we compared the expression levels of ephrin-b ligands in MTLn3-B1 cells and 3T3 cells, as MTLn3-B1 cells failed to undergo CIL when encountering 3T3 cells. 3T3 cells had a decreased expression of ephrin-b ligands as compared with MTLn3-B1 cells ( ∼ 60%, Fig. 5j ), suggesting a threshold of EphB signalling may be necessary to induce CIL. Overall, our results strongly suggest that EphB signalling induces CIL in MTLn3-B1 cells. As CIL signalling induces collapse of leading cell protrusions, we next tested whether exogenously supplied soluble, clustered ephrin-b1-fc could induce protrusion collapse in EGF-stimulated MTLn3-B1 cells. We performed live cell imaging experiments, adding EGF to MTLn3-B1 cells to induce protrusion formation and then subsequently adding either clustered ephrin-b1-fc or clustered fc ( Fig. 6a ). Pre-clustering of exogenous ephrin-fc ligands is needed to induce signalling through Eph receptors [42] . Clustered ephrin-b1-fc induced significant cell retraction while fc treatment had little effect ( Fig. 6b ), suggesting that EphB signalling is functionally sufficient to suppress protrusions generated by EGF stimulation in MTLn3-B1 cells. The suppression of protrusions is likely mediated through inhibition of PI3K, as PI3K activity decreased on the addition of clustered ephrin-b1-fc but showed little change with the addition of clustered fc ( Fig. 6c,d ). 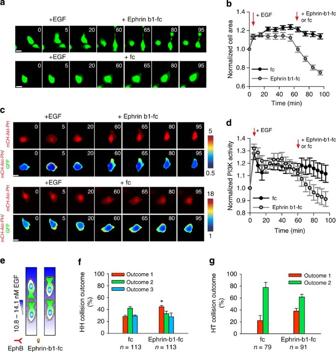Figure 6: EphB signalling suppresses EGF protrusion signalling in MTLn3 Cells. (a) Selected images of MTLn3-B1 cells stimulated with EGF and then treated with either clustered ephrin-b1-fc (top panel) or fc (bottom panel). Green colour indicates expression of GFP. (b) Quantification of cell area after indicated treatments ina. Data are the mean fromn>=90 cells per condition fromn=3 independent experiments. Error bars are s.e.m.. (c) PI3K activity after EGF treatment followed by the addition of either clustered ephrin-b1-fc (top two panels) or fc (bottom two panels). Red colour indicates localization of mCH-Akt-PH, while the pseudocolour indicates the ratio of mCH-Akt-PH to cytosolic GFP. Time is in minutes. Scale bar, 20 μm. (d) Quantification of PI3K activity from data inc. Data are the mean fromn>=22 cells fromn>=3 independent experiments. Error bars are s.e.m. (e) Schematic of EphB receptor masking on incubation with unclustered ephrin-b1-fc ligands. (f,g) HH and HT collision outcome probabilities in 10.8–14.1 nM EGF gradients after preincubation with either 4 μg ml−1unclustered fc or ephrin-b1-fc. Total collisions analysed per condition are displayed. Data are the mean ofn=4 independent experiments per condition. Error bars are s.e.m. Statistical comparisons are made between the same outcome (red bars) in fc versus ephrin-b1-fc using a two-sided Student’st-test. Time is in minutes. Scale bar, 10 μm. *P<.01. Figure 6: EphB signalling suppresses EGF protrusion signalling in MTLn3 Cells. ( a ) Selected images of MTLn3-B1 cells stimulated with EGF and then treated with either clustered ephrin-b1-fc (top panel) or fc (bottom panel). Green colour indicates expression of GFP. ( b ) Quantification of cell area after indicated treatments in a . Data are the mean from n >=90 cells per condition from n =3 independent experiments. Error bars are s.e.m.. ( c ) PI3K activity after EGF treatment followed by the addition of either clustered ephrin-b1-fc (top two panels) or fc (bottom two panels). Red colour indicates localization of mCH-Akt-PH, while the pseudocolour indicates the ratio of mCH-Akt-PH to cytosolic GFP. Time is in minutes. Scale bar, 20 μm. ( d ) Quantification of PI3K activity from data in c . Data are the mean from n >=22 cells from n >=3 independent experiments. Error bars are s.e.m. ( e ) Schematic of EphB receptor masking on incubation with unclustered ephrin-b1-fc ligands. ( f , g ) HH and HT collision outcome probabilities in 10.8–14.1 nM EGF gradients after preincubation with either 4 μg ml −1 unclustered fc or ephrin-b1-fc. Total collisions analysed per condition are displayed. Data are the mean of n =4 independent experiments per condition. Error bars are s.e.m. Statistical comparisons are made between the same outcome (red bars) in fc versus ephrin-b1-fc using a two-sided Student’s t -test. Time is in minutes. Scale bar, 10 μm. * P <.01. Full size image We next investigated how suppression of EphB signalling could affect CIL in chemotaxing MTLn3-B1 cells. Earlier, we showed that enhancing chemotaxis, by overexpressing EGFR or changing input gradients, strongly reduced the probability of CIL ( Fig. 3c , Supplementary Fig 3f ). We hypothesized that suppression of EphB receptor activity would similarly diminish CIL during MTLn3-B1 chemotaxis. Incubation with unclustered ephrin ligands serves as an alternative, complementary approach to inhibiting Eph receptor signalling by saturating receptor binding sites without inducing signalling [42] , [43] ; therefore, we pre-incubated MTLn3-B1 cells with either unclustered fc or ephrin-b1-fc and subsequently induced chemotaxis to gradients of 10.8–14.1 nM EGF (4 μg ml −1 concentration of ephrin-b1-fc or fc Fig. 6e ), the input condition where CIL outcomes previously remained unaffected ( Fig. 3e,j ). We found that CIL outcomes shifted significantly towards Outcome 1 (that is, only the cell migrating away from the gradient undergoes CIL) in HH collisions with ephrin-b1-fc pretreatment versus HH collisions with pretreatment with the fc domain alone ( Fig. 6f ). A similar but smaller shift was seen in HT collisions ( Fig. 6g ). Pretreatment with unclustered ephrin-b1-fc or fc did not significantly affect cell speed in this assay ( Supplementary Fig. 8a ), while reducing the concentration of ephrin-b1-fc (1 versus 4 μg ml −1 ) failed to produce a shift in HH and HT collision probabilities ( Supplementary Fig. 8b,c ), again implying a threshold dependence on EphB signalling for inducing CIL. CIL in 2D assays was also disrupted on pretreatment with unclustered ephrin-b1-fc ( Supplementary Fig. 8d–e ). Taken together, our results suggest that EphB signalling is capable of suppressing MTLn3-B1 cell protrusions arising from EGF stimulation and that perturbation of EphB signalling also alters the balance between CIL and chemotaxis. EphB signalling does not activate RhoA in MTLn3-B1cells Although EphB signalling suppressed EGF-mediated protrusion formation, it was unclear how this suppression was induced. RhoA, a canonical member of the small Rho GTPases, is known to induce contractile signalling [44] and is a downstream mediator of CIL in growth cones [45] , neural crest cells [2] and prostate cancer cells [17] , making it a likely candidate to be activated by EphB signalling. To assess the role of RhoA in EphB signalling in MTLn3-B1 cells, we used a Dora-RhoA FRET reporter (details in Methods) to observe RhoA activity in MTLn3-B1 cells after stimulation with clustered ephrin-b1-fc ( Supplementary Fig. 9a and Supplementary Movie 13 ). Before stimulation, RhoA activity was low and did not increase after the addition of ephrin-b1-fc ( Supplementary Fig. 9a,b ), suggesting that RhoA was not involved in EphB-mediated CIL in MTLn3-B1 cells. Interestingly, individual stimulation with ephrin-b1-fc also did not induce retraction ( Supplementary Fig. 9a,c ), suggesting that EphB signalling may mediate CIL in MTLn3-B1 cells by suppressing protrusive signalling rather than through active contraction. RhoA activity increased and localized to protrusions on the addition of EGF ( Supplementary Fig. 9b,d ), as was previously shown [46] , while a control construct exhibited little change ( Supplementary Fig. 9b,e , Supplementary Movie 13 ). EphB signalling induces CIL via upstream inhibition of PI3K To clarify how EphB signalling inhibits EGF-mediated protrusive signalling, we pretreated MTLn3-B1 cells with clustered ephrin-b1-fc before adding EGF ( Supplementary Fig. 10a ). We hypothesized that EphB signalling would mobilize inhibitory machinery and diminish subsequent EGF-mediated cell spreading. Indeed, we found that pretreatment with ephrin-b1-fc attenuated EGF-induced cell spreading ( Supplementary Fig. 10a,b and Supplementary Movie 14 ), providing evidence that EphB signalling-induced CIL in MTLn3-B1 cells acts through suppression of protrusive signalling. We next focused on identifying where EphB signalling impinges on EGF-mediated protrusive signalling. Earlier, we showed that PI3K was activated in gradients of EGF, maintained persistent activity at leading protrusions, and was inhibited by both cell contact and the addition of ephrin-b1-fc ligands ( Figs 4a,b,f,h and 6c,d ), collectively suggesting that PI3K is inhibited by EphB signalling. However, it remained unclear whether this inhibition occurred directly at or upstream of PI3K. A straightforward method to assess where this inhibition occurs is to directly activate PI3K with and without pretreatment with ephrin-b1-fc. Differences in PI3K-mediated cell spreading after pretreatment with ephrin-b1-fc would suggest that EphB signalling affects PI3K or a molecule downstream of PI3K (such as Rac), while no difference would suggest that EphB signalling inhibits a molecule upstream of PI3K (a logic similar to genetic epistasis analysis). To directly activate PI3K and assess its regulation by EphB, we utilized chemically induced dimerization (CID) [47] , adding rapamycin to localize a PI3K activation construct to the plasma membrane after pretreatment with either clustered ephrin-b1-fc or fc ( Supplementary Fig. 10c and Supplementary Movie 15 ). The presence of rapamycin itself did not alter native PI3K dynamics in MTLn3-B1 cells in response to EGF at this timescale ( Supplementary Fig. 10d ) and therefore could be used to independently alter PI3K activity solely through CID. We did not find any significant differences in MTLn3-B1 cell spreading after induction of PI3K activity with either pretreatment ( Supplementary Fig. 10c,e ), suggesting that EphB-mediated inhibition of EGF signalling occurs upstream of PI3K. To rule out concerns of maximal PI3K activation overriding ephrin-b1-fc-mediated inhibition, we also ran experiments with an order-of-magnitude-lower rapamycin (10 versus 100 nM). We observed a slower, more gradual change in cell area but also did not find any significant differences between clustered ephrin-b1-fc and fc pretreatment ( Supplementary Fig. 10f ). Last, similar experiments conducted for Rac ( Supplementary Fig. 10g,h and Supplementary Movie 16 ) also implied that CIL-mediated interference with chemotactic signalling occurs upstream of this small GTPase. Overall, these results suggest that EphB signalling inhibits EGF-mediated protrusion formation through a mechanism acting upstream of PI3K and Rac activation, at or immediately downstream of the EGF receptor. In vivo directed cell migration often relies on the continuous processing of multiple inputs, instructing a cell to arrest or continue migration, and, importantly, defining the direction of locomotion. The current understanding of how cells integrate and resolve multiple cues is still immature, in spite of important implications for dissecting complex migratory behaviour during processes such as invasion and metastatic spread of tumour cells. Here we explored how cells simultaneously process chemotaxis and CIL cues, both of which play prominent roles in controlling cell migration during metastasis. A controlled direct comparison of these cues at the single-cell level suggests that the direction of migration imparted by one cue can override the other based on a balance between input strengths, suggesting a context-dependent migration cue hierarchy. Controlled manipulations of input conditions can modify directed migration outcomes in a predictable manner, further suggesting a dynamic balance based on the integration of positive (chemotaxis) and negative (CIL) signalling centred at cell protrusions. Our results suggest that both cues act on MTLn3 cells by impinging on a PI3K, Rac and RhoA signalling network, affecting actin polymerization and protrusion formation ( Fig. 7 ). CIL cues are mediated in part by EphB signalling through engagement of ephrin-b ligands present on the surface of other MTLn3 cells, although other repulsive signalling molecules such as N-cadherin, semaphorins and slits could potentially contribute to the induction of CIL. Contrary to previous studies conducted within other cell types, where CIL was induced through RhoA [2] , [17] , we suggest that, in MTLn3 cells, EphB signalling induces CIL through inhibition of EGF-mediated protrusion formation via suppression of PI3K, as the direct addition of clustered ephrin ligands did not activate RhoA and did not induce cell retraction. This idea is further supported by previous work, where EphB signalling was shown to inhibit Akt (a canonical downstream target of PI3K) in non-small-cell lung cancer, resulting in a reduction in chemotaxis without affecting proliferation or apoptosis [48] . Thus, we suggest a different mechanism of CIL induction through suppression of protrusive signalling independent of RhoA and active contractile signalling. 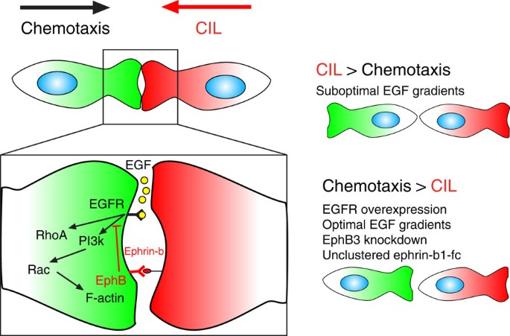Figure 7: Integration of chemotaxis and CIL signalling determines the direction of migration. The interplay between chemotaxis and CIL is mediated in MTLn3-B1 cells by the convergence of EGF (chemotaxis) and EphB/ephrin-b (CIL) signalling above PI3K. Various conditions can shift the signalling balance between pathways and thus affect the resulting direction of migration. Figure 7: Integration of chemotaxis and CIL signalling determines the direction of migration. The interplay between chemotaxis and CIL is mediated in MTLn3-B1 cells by the convergence of EGF (chemotaxis) and EphB/ephrin-b (CIL) signalling above PI3K. Various conditions can shift the signalling balance between pathways and thus affect the resulting direction of migration. Full size image CIL has been described as a driving force for epithelial wound healing, whereby epithelial cells migrate into the free space left by a wound and halt their migration on its closure, commensurate with the re-establishment of contact [49] . The subversion of inherent homotypic CIL mechanisms in advanced epithelial cancers may serve to enhance the overall spread of cancer cells, for example, by preferentially directing individual cells away from the tumour mass. Such interactions could occur in the absence of or distant from chemical gradients through autocrine secretion of migratory cues or other factors in the microenvironment, in close analogy to observations in vivo in Cajal–Retzius cells [43] and haemocytes [50] , which are initially clustered cell populations but form uniform cell distributions across their locales after extensive CIL interactions. Scattered cancer cells would thus have an increased probability of finding sources of chemical gradients from exit targets, such as blood vessels. Once these chemical gradients are detected, chemotaxis would serve as a potent cue in eliciting a strong directional migration response. Responsiveness to both CIL and chemotaxis may thus be mutually beneficial in enhancing the directed migration of cancer cells during metastasis. Potential complications may arise when strong chemotactic and CIL cues are present simultaneously, as collisions between chemotaxing cells could redirect them away from their intended targets and reduce overall chemotactic efficiency. We find that, in the presence of potent chemical gradients, cells migrating up gradients have a significantly decreased probability of undergoing CIL. This decrease is mediated through two complementary mechanisms, re-establishment of polarity in the original direction following protrusion collapse and having more stable protrusions which are unaffected by cell contact. The suppression of CIL during chemotaxis further allows contacting cells to migrate as clusters, suggesting that growth factors or other pro-migratory extracellular cues can induce a transition from an individual cell migration mode into more collective migration, in the context of CIL. CIL could also serve as a way for cells to evaluate the strength of chemotactic gradients, as only sufficiently strong chemotactic inputs can be effective in overcoming CIL. Overall, our results suggest a complex interplay between CIL and chemotactic cues that are reflective of the ability of single live cells to perform effective decision making while presented with potentially conflicting inputs. Cell culture and reagents MTLn3 GFP, MTLn3-B1 GFP and MTLn3-B1 cells were a gift from J. Segall (Albert Einstein College of Medicine, NY). MTLn3 GFP, MTLn3-B1 GFP and MTLn-B1 cells were maintained in αMEM (Cellgro) with 5% FBS (Gibco) and 1% penicillin/streptomycin (Sigma). 3T3 cells (NIH/3T3) were a gift from J. Zhang (Johns Hopkins School of Medicine, MD) and were cultured in DMEM (Cellgro) with 10% FBS (Gibco) and 1% penicillin/streptomycin. All cell lines were cultured in a humidified 37 °C and 5% CO 2 incubator. EGF (PHG0311), Rat tail collagen 1 (A1048301) and IgG1-fc (10702HNAH50) were obtained from Life technologies. Ephrin-fc ligands (SMPK3) and E-cadherin-fc (748-EC-050) were obtained from R&D systems. Rapamycin (R-5000) used in CID experiments was from LC laboratories. The following primary antibody was used for immunostaining-rabbit monoclonal anti-E-Cadherin IgG (Cell Signaling, 3195), while the following primary antibodies were used for western blotting-rabbit monoclonal anti-EphB3 IgG (Abcam, ab133742), rabbit polyclonal ephrin-b1/b2/b3 IgG (Santa Cruz, sc-910) and mouse monoclonal anti-GAPDH IgG (Santa Cruz, sc-32233). The following secondary antibodies were used: Goat anti-human IgG fc (109-005-098) (Jackson ImmunoResearch), FITC-conjugated Goat anti-human IgG fc (AP113F) (Millipore), Alexa Fluor 594 Goat anti-rabbit IgG (Life technologies, A-11012), ECL rabbit HRP-linked IgG (GE healthcare, NA934) and ECL mouse HRP-linked IgG (GE healthcare, NA931). Transfections were carried out using Fugene HD (Promega) according to the manufacturer’s recommendation. MTLn3-B1 cells without GFP expression were used for all FRET experiments. For direct activation experiments, YFP-FKBP-iSH (PI3K activation construct) and YFP-FKBP-Tiam1 (Rac activation construct) were co-transfected with Lyn 11 -FRB (LDR) into MTLn3-B1 cells without GFP expression. The Raichu-Rac FRET construct was a gift from M. Matsuda (Tokyo University, Japan). The Dora-RhoA sensor was constructed based on the design principle developed previously [51] , [52] . To improve dynamic range, structural optimization was incorporated in the sensor to couple dimerization of fluorescent protein with RhoA activation, hence the name dimerization optimized reporter for activation (Dora). As a result, it contains a RhoA-binding domain of PKN at the N terminus (S14-H97) that is circularly permutated (at R68-S69), followed by a fluorescent protein FRET pair (Cerulean3 circularly permutated Venus) that is connected with repeats (3 × ) of helical linker (EAQKQKEQRQAAEELAN) derived from the ribosomal protein L9 (ref PMID 9245593) and, an intact, wild-type RhoA at the C terminus. The detailed development and characterization of the sensor will be described elsewhere. As a control, a point mutation (L59Q) was introduced in the RhoA-binding domain of PKN in the sensor to disrupt RhoA binding. While the RhoA in the mutant construct remains capable of interacting with its regulatory proteins, the mutant sensor controls for potential alterations of FRET signals in the cell that are independent of RhoA activation. Device fabrication Microfluidic devices were fabricated using a traditional two-layer soft lithography process [53] out of polydimethylsiloxane (PDMS, RTV615) from Momentive by replica moudling off of silicon wafer masters. Silicon masters were created using standard photolithography techniques [54] . Device designs were created in Freehand MX (Macromedia) and AutoCAD (Autodesk). Device protocol The microfluidic device was designed to simultaneously generate a gradient across all cells at the same time. To achieve this design goal, we surrounded the microchannels with an intermediate rounded zone, accessible to built-in elastomeric valves from above ( Supplementary Fig. 1c ). Pressurizing the valves causes the rounded zones to collapse, effectively isolating the microchannels from the source and sink. In this manner, the source and sink can be pre-established at steady state around the microchannels without transient stimulation, thus ensuring all microchannels receive the gradient coincidently when the valves are released ( Supplementary Fig. 1b,c ). Gradients reach steady state in ∼ 10 min and can be maintained for >8 h ( Supplementary Fig. 1b ). We used device simulations to calculate the effect of including the rounded zone on gradient production and found that the effective gradient across the microchannels was 30–70% of the source value ( Supplementary Fig. 1d,e ). Microfluidic devices were prepared by cleaning with 70% ethanol and an alconox solution. Devices were then bonded to 22 × 40 mm #1.5 coverglass (Fisher) and incubated in an oven set at 80 °C overnight. Before experiments, device valves were first filled with DI water by pressurizing with 10 PSI using solenoid valves (The Lee company). Subsequently, valves ‘5’ and ‘7’ (Shown in blue, Supplementary Fig. 1a ) were pressurized to restrict fluid flow to the gradient generation region and a 40 μg ml −1 collagen 1 solution was introduced into one of the two ‘c’ ports (shown in green, Supplementary Fig. 1a ) to fill the source, sink and microchannel region. Devices were coated with collagen for 1 h before the collagen solution was exchanged for cell medium. Cells were seeded as follows: cells were trypsinized and resuspended in normal cell culture medium at a concentration of 10 million cells ml −1 . The cell suspension was then pipetted onto one of the ‘c’ ports and induced into the microchannel region by gravity flow. To terminate cell seeding, the valve opposite to where cells were introduced was pressurized (either valve ‘6’ or valve ‘8’) and the pressure in valve ‘5’ was released to allow extraneous cells to be removed from the source and sink channels via flow from the inlet labelled ‘w’ (shown in red, Supplementary Fig. 1a ). Cells were allowed to adhere for 3–4 h before experimentation. Typical experiments were run with cell medium solution in the sink side of the device and an EGF-containing solution in the source side. Input solutions were introduced from the inlet network labelled ‘1–4’ (shown in green, Supplementary Fig. 1a ). During the establishment of the source and sink, cells in the microchannel region were isolated by pressurizing valves ‘8’ and ‘6’ ( Supplementary Fig. 1c ). Finally, experiments were initiated when these valves were released and gradients of EGF were allowed to form across the microchannels via diffusion between the pre-established source and sink ( Supplementary Fig. 1c ). In experiments where MTLn3-B1 cells were pretreated with ephrin-b1-fc or fc, solutions with either 4 μg ml −1 ephrin-b1-fc or fc were introduced into the device from the ‘w’ inlet while cells were isolated by pressurizing valves ‘8’ and ‘6’. After fluid exchange within the device to ephrin-b1-fc or fc, the valves were released and cells were pretreated for 45 min before experimentation. Imaging Live cell imaging experiments were performed on a Zeiss Axiovert 200 M epifluorescence microscope with a motorized stage (Prior) in an environmental chamber (Pecon) set at 37 °C and 5% CO 2 with a 40X, 1.3 numerical aperture oil immersion objective (Zeiss) coupled to a Cascade II:1024 EMCCD camera (Photometrics). Slidebook software (Intelligent Imaging Innovations) was used for automated control of the microscope system. Immunostained samples were imaged on a confocal Zeiss LSM510-Meta using a 63X Planapo oil objective driven by Zen software (Zeiss). Live cell imaging experiments MTLn3 cells were seeded onto acid washed 25-mm glass coverslips (Fisher) coated with 40 μg ml −1 Rat Tail Collagen 1 for 1 h at room temperature. Cells were allowed to attach overnight and then were subsequently starved for 3 h in L15 medium with 0.35% BSA (Life Technologies). The glass coverslip was then transferred to Attofluor live cell imaging chambers (Life Technologies), mounted onto the microscope and stimulated with 100 ng ml −1 EGF or 1 μg ml −1 preclustered ephrin-b1-fc. Ephrin-b1-fc was preclustered with a 1/10 concentration of Goat anti-human fc for 1 h at 37 °C. In some experiments, EGF treatment was followed by the addition of 1 μg ml −1 preclustered ephrin-b1-fc or 1 μg ml −1 preclustered fc. Chemically induced dimerization Chemically induced dimerization refers to a well-established set of techniques to manipulate endogenous signalling without receptor activation through spatial-temporal control over rapamycin-mediated association between FK506-binding protein (FKBP) and the FKBP–rapamycin-binding domain (FRB) [21] , [55] . To active PI3K, we applied rapamycin to localize a previously developed PI3K activation construct [55] , consisting of a PI3K activator (interSH2), a fluorescent protein (YFP) and FKBP, with membrane-anchored FRB. To activate Rac, we applied rapamycin to localize a YFP-FKBP-tagged Rac GEF (Tiam1) to the plasma membrane-anchored FRB. Image analysis and metrics Image analysis was carried out using custom scripts written in Matlab 2007b (Mathworks). All images were first flatfield and darkfield corrected using the following routine: C=(I−D/F−D) × M where C=corrected image, I=initial image, D=darkfield image, F=flatfield image, and M=mean of difference between flatfield and darkfield images. Flatfield and darkfield images were obtained by averaging multiple images. Images were then background subtracted and Gaussian filtered to remove noise. To analyse cell speed and the chemotaxis index, cells were semi-automatically segmented by thresholding from GFP images and position data were generated by obtaining the centroid of segmented cells. Only cells that did not come into contact with other cells were used in this analysis. The chemotaxis index is defined as the distance moved up the gradient divided by the total distance travelled. Positive values were given to migration up the gradient, while negative values were given to migration in the opposite direction. To analyse mCherry-Akt-PH biosensor data, cell images were background subtracted and then segmented by thresholding from mCherry images to create a binary mask. This mask was then multiplied into both the original mCherry image and the GFP image to isolate the fluorescence data of a single cell. The single-cell mCherry image was then divided by the single-cell GFP image to obtain the ratio. In experiments performed in open chambers, PI3K activity was averaged from the cell perimeter. The cell perimeter was isolated by using a morphological erosion on the binary mask produced from segmentation of the mCherry-Akt-PH image and subtraction of this image from the original binary mask. To analyse FRET data (Raichu-Rac, Dora-RhoA), we followed a previously described protocol [56] . In brief, CFP and YFP FRET images (CFP excitation, YFP emission) were background subtracted, thresholded based on intensity and aligned with a dft registration algorithm. The final ratio images were obtained by dividing the YFP FRET image by the registered CFP image. Final ratio images were Gaussian filtered. FRET data from Dora-Rhoa were obtained by taking a whole-cell average from the ratio image. The polarization ratio in microfluidic experiments was obtained by segmenting ratio images into binary images. Rows of the resulting binary images were then used to define the cell length. The polarization ratio was then obtained by taking the ratio between the mean value of the front 20% of the cell length and the rear 20% of the cell length from the original ratio images. We define front as where a protrusion is generated. CIL outcomes in microfluidic experiments were analysed by observing GFP time series and assessing the direction of migration within 60 min post collision, as this was the longest observed duration for resolving CIL in uniform EGF ( Supplementary Fig. 4a ). Cells that either reformed protrusions in the original direction of their migration post collision or whose protrusions remained unaffected were considered to have not undergone CIL. In HH collisions, we observed a few rare events where cells lost polarity and remained unpolarized for a significantly longer duration than 60 min as a result of cell division or other cellular phenomena. Such events were excluded from analysis. In HT collisions, we considered cells that were not redirected in 60 min as Outcome 1 based on the same rationale as above. CIL in 2D was analysed using a previously described metric [17] , [18] by tracking cell positions 60 min before and after cell collisions. Cell areas were analysed by segmenting cells from GFP or YFP images (dimerization experiments). Only cells that did not contact other cells were used in this analysis. Immunostaining For live cell immunostaining, MTLn3-B1 cells were seeded onto collagen-coated glass coverslips and allowed to attach overnight. Cells were subsequently starved for 3 h and incubated with either 1 μg ml −1 unclustered ephrin-fc or fc for 5 min at 37 °C. Next, cells were washed thrice with cold starvation medium and then incubated with a FITC-conjugated Goat anti-human IgG fc antibody (1:100) on ice for 1 h. Finally, cells were washed thrice in starvation medium, fixed for 15 min in 1% paraformaldehyde (Sigma) with Hoechst 33342 (1:500) (Sigma), washed twice in PBS and mounted onto glass slides (Fisher) with ProLong Antifade (Life Technologies). All other immunostaining was carried out as follows: MTLn3-B1 cells were seeded onto collagen-coated glass coverslips and allowed to attach overnight. Cells were subsequently starved for 3 h and fixed for 25 min in 4% PFA, permeabilized in 0.1% Triton for 7 min, blocked with 10% Goat serum in PBS for 1 h, incubated with primary antibodies (1:200) for 1 h, incubated with secondary antibodies with Hoechst 33342 (1:500) for 1 h and then mounted onto glass coverslides with ProLong. PBS washes were carried out in between steps. Western blotting MTLn3-B1 cells and 3T3 cells were grown to 80% confluence before harvesting. In siRNA experiments, MTLn3-B1 cells were transfected for 48 h before harvesting. To create cell lysates, cells were washed in cold PBS followed by lysis in RIPA (Thermo scientific) with protease/phosphatase inhibitors (Thermo scientific) and were subsequently sonicated (Qsonica) and spun down. Lysates were incubated with loading buffer and separated by sodium dodecyl sulfate–PAGE (SDS–PAGE) using pre-cast 4–12% Bis Tris Gels (Life Technologies) and were transferred to nitrocellulose membranes using an iBlot system (Life Technologies) for subsequent probing and imaging using ECL (Pierce). The following antibody dilutions were used: anti-EphB3 (1:1,000), anti-ephrinb1/b2/b3 (1:250), anti-GAPDH (1:1,000), anti-Rabbit HRP linked (1:2,000) and anti-Mouse HRP linked (1:10,000). Western blot images were quantified using ImageJ. All bands were normalized to a loading control (GAPDH). Uncropped blots are in Supplementary Fig. 11 . siRNA MTLn3-B1 cells were transfected with 100 nM siRNA using Oligofectamine (Life technologies) for 4 h in serum-free medium. The transfection was terminated by adding 2 × serum-containing medium and cells were incubated for ∼ 48 h befor experimentation. A set of 4 ON-TARGET plus siRNAs against rat EphB3 (EphB3 siRNA #1- 5′- AGAGCAAGACUAUCGGUUA-3′, EphB3 siRNA #2- 5′-CGAAAUGGGUGACGUCCGA-3′, EphB3 siRNA #3- 5′-CCAAUGAGGCCGUCCGAGA-3′, EphB3 siRNA #4- 5′-GGACCUUGGCGGACGAGAU-3′) and a non targeting siRNA (5′-UGGUUUACAUGUCGACUAA-3′) was obtained from Dharmacon (LQ-087421-02-0002, D-001810-01-05). EphB3 siRNA#1 was used for knockdown experiments. Mock cells were treated with Oligofectamine without siRNA. Bead preparation The 5-μm protein A-coated silica beads were obtained from G. Kisher (PSi-5.0 PA). To coat beads, either 50 μg ml −1 fc or ephrin-fc was incubated with 1 μl of beads for 1 h at room temperature under agitation. After coating, beads were centrifuged and washed thrice with PBS+1% BSA to remove weakly bound ligands and left in 4 °C under gentle agitation overnight. The protein concentration in the solutions containing ephrin-fc or fc was measured using a nanodrop (Thermo Scientific) before and after the addition of beads to confirm that beads were coated. Real-time RT-PCR MTLn3 cells were harvested from cell culture dishes using RNA protect (Qiagen). An RNeasy Plus kit (Qiagen) was then used to extract RNA from MTLn3-B1 cells. cDNA was created using a Quantitect Reverse transcription kit (Qiagen). Real-time RT-PCR assays were carried out on a Quantstudio system (Applied Biosystems) using Taqman gene expression assays with a Taqman gene expression mastermix (Life Technologies). The following Taqman primers designed for rat were used and obtained from Life Technologies: β-actin (Rn00667869_m1), ephrin-b1 (Rn00438666_m1), ephrin-b2 (Rn01756899_m1), EphB1 (Rn01446845_m1), EphB2 (Rn01181017_m1), EphB3 (Rn01404119_m1), EphB6 (Rn01456014_g1). All results were normalized to β-actin from the same well. Each experiment was carried out in quadruplicate in three independent biological replicates. Statistical analysis Statistical comparisons were carried out in SigmaPlot (Systat). If assumptions of normality were fulfilled (as assessed with a Shapiro-Wilk test), comparisons were made with a two-sided t -test. If assumptions of normality or equal variance were not satisfied, a Mann–Whitney rank sum test was utilized. P values <0.05 were deemed to be significant. How to cite this article: Lin, B. et al. Interplay between chemotaxis and contact inhibition of locomotion determines exploratory cell migration. Nat. Commun. 6:7619 doi: 10.1038/ncomms7619 (2015).